Sgs1 and Sae2 promote telomere replication by limiting accumulation of ssDNA In budding yeast, DNA ends are processed by the consecutive action of MRX/Sae2 and two redundant pathways dependent on Sgs1/Dna2 and Exo1, and this processing is counteracted by Ku heterodimer. Here we show that DNA end resection by Sae2 and Sgs1 is dispensable for normal telomere maintenance by telomerase. Instead, these proteins facilitate telomere replication and limit the accumulation of single-strand DNA (ssDNA) at replication fork pause sites. Loss of Sae2 and Sgs1 drives selection for compensatory mutations, notably in Ku, which are responsible for abrupt telomere shortening in cells lacking Sae2 and Sgs1. In telomerase-negative cells, Sae2 and Sgs1 play non-overlapping roles in generating ssDNA at eroded telomeres and are required for the formation of type II survivors. Thus, although their primary function in telomerase-positive cells is to sustain DNA replication over the sites that are prone to fork pausing, Sae2 and Sgs1 contribute to telomere resection in telomerase-deficient cells. In budding yeast, DNA double-strand breaks (DSBs) are primarily repaired by homologous recombination (HR), whereas non-homologous end-joining (NHEJ) plays minor role. Exonucleolytic degradation of the 5′ end of a DSB is the first and decisive step that channels repair to HR. The MRX (Mre11/Rad50/Xrs2) complex is recruited to the break shortly after it is formed and cooperates with Sae2 to initiate end resection. Extensive resection is then dependent on the 5′–3′ exonuclease Exo1 and on the concerted action of the Sgs1/Top3/Rmi1 complex with the Dna2 endonuclease [1] , [2] , [3] , [4] . In contrast to DSBs, natural chromosome ends are shielded from the action of the DNA damage checkpoints (CPs) and DNA repair pathways by telomeres. Telomeres consist of a tandem array of short repeated sequences, rich in guanines that vary in length and sequence from organism to organism and are bound by a set of specific proteins involved in both telomere length regulation and DNA end protection. In the budding yeast Saccharomyces cerevisiae , the chromosome ends contain 250–350 bp duplex DNA arrays of TG 1–3 repeats and terminate in a 10–15 base extension of the G-rich strand [5] , [6] . At least three different complexes contribute to the capping function and prevent telomeres from being recognized as DSBs: Rap1-Rif1-Rif2 bound to double-stranded telomeric repeats [7] , [8] , the CST (Cdc13, Stn1, Ten1) complex that covers the G-tail [9] , [10] , [11] and the Ku heterodimer that directly binds to the terminal telomeric DNA [12] , [13] . One role of these complexes is to control the action of the nucleases/helicases involved in DSB resection [14] . In late S-phase, the length of telomeric single-stranded G-tails increases transiently from 10–15 to about 30–50 nucleotides [15] . G-tail formation is thought to result from the 5′ end resection of the C-rich strand rather than elongation of the 3′ overhang by telomerase [16] . The resection is initiated by the combined action of MRX and Sae2 (refs 17 , 18 ). As for DSB, the initial overhang is further processed by Sgs1-Dna2 and Exo1, but at native telomeres, Exo1 activity is limited by yKU70/80 and CST thereby confining the extension of resection [17] , [19] , [20] , [21] , [22] . On the other hand, the action of Rap1/Rif2 limits MRX binding at de novo telomeres [23] , [24] , whereas Rap1/Rif1 supports the protection function of the CST complex by a yet unknown mechanism [25] . The MRX complex also plays a key role in targeting telomerase to short telomeres [26] by recruiting Tel1 via specific interaction with a conserved motif in the Xrs2 C-terminus [26] , [27] , [28] . Finally, owing to a high GC content and the presence of stable protein/DNA complexes, telomeres are a challenge for the replication machinery that might become dependent on a specific set of proteins to avoid fork collapse in telomeric repeats [6] , [29] . In the absence of telomerase, telomere erosion leads to replicative senescence [30] . Although the signal of senescence is not fully understood, it is believed that short telomeres lose their capping function and are subject to unregulated degradation by nucleases. Accordingly, the amount of single strand DNA increases at telomeres during senescence [31] and RPA is increasingly recruited to telomeres in parallel with the loss of viability of senescing cells [32] . Interestingly, the recruitment of RPA in regions adjacent to telomeres increases at the peak of senescence suggesting that degradation of the 5′ strand reaches subtelomeric regions [32] . Surprisingly, deletion of EXO1 hardly affects the rate of senescence in the absence of telomerase [20] . The sgs1 Δ mutation also has a counter-intuitive phenotype in telomerase-deficient cells, as it leads to an accelerated senescence, although Sgs1 participates with Exo1 in the degradation of the 5′ strand at uncapped telomeres [33] , [34] . This apparent discrepancy could be explained by the accumulation of recombination intermediates in sgs1 Δ tlc1 Δ cells during senescence, pointing out multiple roles of Sgs1 at telomeres [35] . Previous work established that 5′ end resection at S. cerevisiae telomeres is primarily controlled by consecutive action of Sae2 and Sgs1 (ref. 17 ). In addition, native telomeres are dramatically short in sae2 Δ sgs1 Δ cells. These findings argue for the dependence of telomerase activity on Sae2- and Sgs1-controlled generation of the 3′ overhang [17] . In this study, we examined the function of Sae2 and Sgs1 at native telomeres in both telomerase-proficient and -deficient cells. Our data show that telomeres can be maintained at wild-type (WT) length by telomerase in sae2 Δ sgs1 Δ cells. We explain that the short telomeres in sae2 Δ sgs1 Δ are due to the acquisition of point mutations, notably in yKu. Our results indicate that the primary function of Sae2 and Sgs1 in telomerase-positive yeast is to facilitate telomere replication. In telomerase-negative cells, Sae2 and Sgs1 promote telomere erosion, but this function does not appear to be essential for telomere elongation by telomerase. Abrupt shortening of native telomeres in sae2Δ sgs1Δ cells To clarify the origin of short telomeres in sae2 Δ sgs1 Δ double mutant [17] , we examined telomere length dynamics during expansion of colonies obtained from the sporulation of a SAE2/sae2 Δ SGS1/sgs1 Δ heterozygous diploid strain. In our strain background, about 70% of the s ae2 Δ sgs1 Δ spores were viable ( Supplementary Fig. 1a ). s ae2 Δ sgs1 Δ spore colonies were grown in rich liquid medium and were propagated by diluting saturated cultures every 2 days. Initial telomere length was nearly WT in all clones, but after the second or third subculturing it dropped abruptly from 300 to about 150 bp in the majority of the clones (75%, n =60; Fig. 1a , pattern I). These short telomeres were then maintained at a new length setting without apparent change throughout the generations. In rare instances (2 out of 60), telomeres that were abruptly shortened returned to WT ( Fig. 1a , pattern II). Finally, for about 20% of the clones, telomere length was maintained at a constant length throughout the experiment ( Fig. 1a , pattern III). 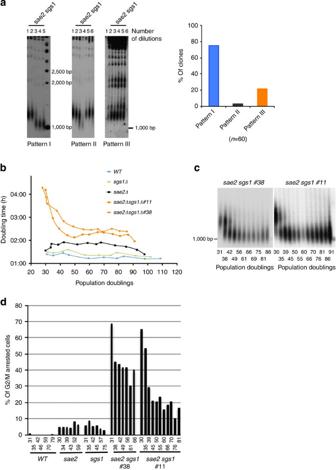Figure 1: Abrupt telomere shortening insae2Δsgs1Δ cells. (a)sae2Δsgs1Δ spore colonies obtained from the dissection of a heterozygous diploid were transferred to 2 ml of YPD liquid medium and grown to saturation (about 30 PDS from the original spore, d1). This starting culture was diluted every 2 days to OD600=0.01 into fresh medium (dilutions 2–5). Telomere length was analysed by TG1–3probed Southern blot ofXhoI-digested genomic DNA isolated at each time point. A representative clone for each pattern and quantification of the different patterns of telomere length dynamics (right graph,n=60) are shown. (b) Freshly isolated spore colonies with the indicated genotypes were maintained as exponentially growing cultures in liquid YPD medium for about 100 generations. Doubling times were monitored by measuring OD600. (c) Aliquots of cells were taken about every five generations to analyse telomere length. (d) The percentage of G2/M-arrested cells was monitored by microscopic analysis of cell morphology at each time point. Figure 1: Abrupt telomere shortening in sae2 Δ sgs1 Δ cells. ( a ) sae2 Δ sgs1 Δ spore colonies obtained from the dissection of a heterozygous diploid were transferred to 2 ml of YPD liquid medium and grown to saturation (about 30 PDS from the original spore, d1). This starting culture was diluted every 2 days to OD 600 =0.01 into fresh medium (dilutions 2–5). Telomere length was analysed by TG 1–3 probed Southern blot of Xho I-digested genomic DNA isolated at each time point. A representative clone for each pattern and quantification of the different patterns of telomere length dynamics (right graph, n =60) are shown. ( b ) Freshly isolated spore colonies with the indicated genotypes were maintained as exponentially growing cultures in liquid YPD medium for about 100 generations. Doubling times were monitored by measuring OD 600 . ( c ) Aliquots of cells were taken about every five generations to analyse telomere length. ( d ) The percentage of G2/M-arrested cells was monitored by microscopic analysis of cell morphology at each time point. Full size image Growth in liquid medium of two representative sae2 Δ sgs1 Δ spore clones with pattern I is shown ( Fig. 1b ). We measured the number of population doublings (PDs) while maintaining cells in log-phase by consecutive dilutions. At the first time point, sae2 Δ sgs1 Δ cells that had undergone approximately 30 PDs from the original spore grew poorly with a doubling time of about 4.5 h. The doubling time, however, decreased at least twofold after about 40–50 PDs ( Fig. 1b ). Microscopic observation of the cell cycle distribution of sae2 Δ sgs1 Δ cells showed that about 70% of the freshly isolated sae2 Δ sgs1 Δ cells displayed a dumbbell-shape with the nucleus at, or spanning, the neck typically found in G2-arrested cells ( Fig. 1d ). This percentage dropped to about 20–40% concomitantly with the appearance of short telomeres and was maintained at this level throughout the subsequent generations ( Fig. 1c,d ). We concluded that sae2 Δ sgs1 Δ cells with WT length telomeres experience chronic CP activation indicative of an accumulation of aberrant DNA structures. CP activation appeared to be essential for the survival of sae2 Δ sgs1 Δ cells, as we were unable to isolate viable sae2 Δ sgs1 Δ mec1 Δ sml1 Δ mutants. The apparent rate and mode of telomere shortening displayed by pattern I were incompatible with the average replicative loss of 4–5 bp per PD that is observed when telomerase activity is defective. Therefore, a mechanism other than impaired telomerase activity likely is involved in generation of the short telomeres. Spontaneous yku mutations in sae2 Δ sgs1 Δ liquid cultures Because deletion of yKU was shown to rescue sae2 Δ and sae2 Δ sgs1 Δ defects and to cause an acute shortening of telomeres [36] , [37] , [38] , we sequenced YKU70 and yKU80 in five independent clones showing pattern I ( Fig. 2 ). Although at t1 (about 30 PDs), all clones had WT yKU70 and yKU80 , four out of five clones exhibited point mutations in either yKU70 or yKU80 at t3 ( Table 1 ). yku70 -L38Q, yku80 -C410F,A410S and yku80 -Y495D map onto the human Ku structure [39] within the N-terminal α/β domain, β-barrel and C-terminal arm, respectively. yKu70- V570G is located in a region predicted to be the last α-helix of the protein. Strikingly, the mutation yku70 -L38Q was also obtained ( yKu70-1 ) in a screen aimed to identify Ku mutants that bypass the requirement for Mre11 nuclease activity in the repair of camptothecin-induced DNA lesions; and the yku80 -Y495D mutation is nearly symmetrical to the Y494N mutation ( yKu70-5 ) identified in the same screen [40] . We found that all ku70 and ku80 mutant alleles partially rescued the growth of ku70 Δ and ku80 Δ strains at 37 °C, but they all had reduced telomere length ( Supplementary Figs 2a,b ). 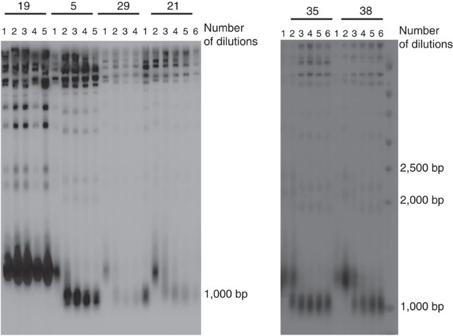Figure 2:sae2Δsgs1Δ cells acquire suppressive mutations inYKU. Telomeres length analysis of six independentsae2Δsgs1Δ clones maintained in liquid culture by serial dilutions as described inFig. 1a. The genes for both subunits of the Ku heterodimer were sequenced for each clone. The point mutations associated with abrupt telomere shortening are given inTable 1. Figure 2: sae2 Δ sgs1 Δ cells acquire suppressive mutations in YKU. Telomeres length analysis of six independent sae2 Δ sgs1 Δ clones maintained in liquid culture by serial dilutions as described in Fig. 1a . The genes for both subunits of the Ku heterodimer were sequenced for each clone. The point mutations associated with abrupt telomere shortening are given in Table 1 . Full size image Table 1 YKU70 and YKU80 sequence analysis. Full size table Taken together, these results suggest that both rescue of the slow growth and abrupt telomere shortening are the consequences of the strong selection for yku mutants in the s ae2 Δ sgs1 Δ background. Mapping of the yku mutations on the human Ku structure [39] showed that they occurred in the structural elements important for DNA binding. It is likely that these yku mutants exhibit reduced affinity for DNA ends, as do those described by Petrini and colleagues [40] . If the basis of suppression of sae2 Δ sgs1 Δmutant phenotype by yku mutations is to restore end resection by allowing Exo1 access to DSBs arising during DNA replication [36] , [37] , [40] , [41] , then the rescue should be dependent on HR. We found that deleting RAD52 reduced the size of the sae2 Δ sgs1 Δ yKu70Δ spore colonies ( Supplementary Fig. 3a ). In line with this, there was no selection for y KU mutation in sae2 Δ sgs1 Δ cultures in the absence of RAD52 as none of the rad52 Δ sae2 Δ sgs1 Δ clones we analysed displayed abrupt telomere shortening. Instead, telomere length remained about WT for up to 100 PDs in this genetic context ( Fig. 3a ). We then asked whether telomere loss in sae2 Δ sgs1 Δ cells could be also prevented in the absence of Rad51 and Rad59 that define two distinct pathways of Rad52-dependent HR [42] . Out of the 34 independent sae2 Δ sgs1 Δ rad59 Δ clones analysed, 35% (instead of 76% in the sae2 Δ sgs1 Δ clones, P =0,00013) showed an abrupt telomere shortening after about 40 PDs, whereas telomeres remained at a stable WT length in the other clones ( Fig. 3b ). In contrast, deletion of RAD51 did not prevent shortening of telomeres in most of the clones analysed ( Fig. 3b ). This suggests that Rad59 rather than Rad51 functions together with Rad52 to promote growth of sae2 Δ sgs1 Δ cells in the absence of a fully functional Ku complex. 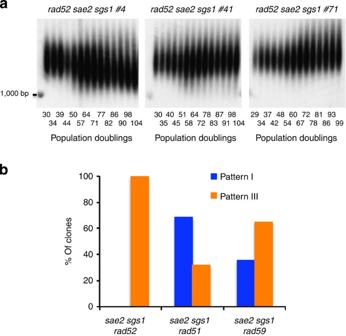Figure 3: Telomerase is active insae2Δsgs1Δ cells. (a) Freshly isolatedrad52Δsae2Δsgs1Δ spore colonies were maintained as exponentially growing cultures in liquid YPD medium for about 100 generations. Aliquots of cells were taken about every five generations to analyse telomere length. (b) Freshly isolated triple mutant clones of the indicated genotypes were transferred to 2 ml YPD liquid medium, grown to saturation and diluted every 2 days. Telomere length was analysed at each time point by TG1–3probed Southern blots and the clones classified as pattern I, II, III according to telomere length dynamics. No clone with pattern II was observed in this experiment.sae2Δsgs1Δrad52Δ (n=15),sae2Δsgs1Δrad59Δ (n=34),sae2Δsgs1Δrad51Δ (n=22). Figure 3: Telomerase is active in sae2 Δ sgs1 Δ cells. ( a ) Freshly isolated rad52 Δ sae2 Δ sgs1 Δ spore colonies were maintained as exponentially growing cultures in liquid YPD medium for about 100 generations. Aliquots of cells were taken about every five generations to analyse telomere length. ( b ) Freshly isolated triple mutant clones of the indicated genotypes were transferred to 2 ml YPD liquid medium, grown to saturation and diluted every 2 days. Telomere length was analysed at each time point by TG 1–3 probed Southern blots and the clones classified as pattern I, II, III according to telomere length dynamics. No clone with pattern II was observed in this experiment. sae2 Δ sgs1 Δ rad52 Δ ( n =15), sae2 Δ sgs1 Δ rad59 Δ ( n =34), sae2 Δ sgs1 Δ rad51 Δ ( n =22). Full size image Telomerase maintains WT telomere length in sae2 Δ sgs1 Δ As described above, in none of the sae2 Δ sgs1 Δ rad52 Δ clones, we observed the progressive decrease of telomere length typical of telomerase dysfunction ( Fig. 3a ). To get insight into the type of telomeric events that occur in sae2 Δ sgs1 Δ cells, we used telomere PCR [43] to sequence a subset of telomeres from a single chromosome end from a population of cells grown for 30 PDs of clonal expansion. Yeast telomerase adds imperfect repeats of the sequence TG 1–3 . As a consequence, after clonal outgrowth, telomere shortening and elongation can be detected via the divergence of telomeric sequences in telomere distal region, which is maintained by telomerase, whereas the proximal sequences remain unchanged [43] . Telomeres from two independent clones of each WT and sae2 Δ sgs1 Δ cells were sequenced after 30 PDs ( Fig. 4 ). Notably, the frequency of telomere sequence divergence was similar in WT and sae2 Δ sgs1 Δ cells after 30 PDs ( Fig. 4 and Table 2 ), but the mean length of the divergent sequences was greater in the double mutant, especially when the point of divergence was under 250 bp. Therefore, either telomerase is more processive in double mutant or there is a contribution of recombination. To resolve this issue, we sequenced telomeres from the sae2 Δ sgs1 Δ rad52 Δ cells. No significant difference was detected between the triple mutant and WT cells ( Table 2 ). We concluded that telomeres can be maintained by telomerase alone in sae2 Δ sgs1 Δ cells, but recombination also contributes to elongate telomeres in these cells. 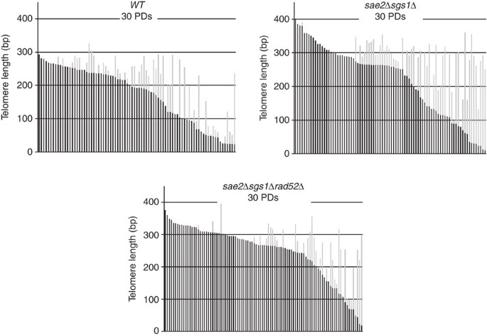Figure 4: Enhanced TG1–3repeat extension insae2Δsgs1Δ cells. Cells of the indicated genotypes were isolated from heterozygous diploids and grown for the indicated number of population doublings (PDs). Telomere at the left arm of chromosome I (TEL01L) was amplified by PCR, cloned and sequenced from two independent clones for each genotype. Individual telomeres are represented by vertical bars with the conserved centromere-proximal sequence in black and the distal divergent sequence in grey, and ordered according to the length of the conserved sequence. Figure 4: Enhanced TG 1–3 repeat extension in sae2 Δ sgs1 Δ cells. Cells of the indicated genotypes were isolated from heterozygous diploids and grown for the indicated number of population doublings (PDs). Telomere at the left arm of chromosome I (TEL01L) was amplified by PCR, cloned and sequenced from two independent clones for each genotype. Individual telomeres are represented by vertical bars with the conserved centromere-proximal sequence in black and the distal divergent sequence in grey, and ordered according to the length of the conserved sequence. Full size image Table 2 Telomere sequence analysis. Full size table We next asked whether telomerase activity is sensitive to the negative regulation by Rif2, which competes with Tel1 binding at telomeres [27] , [44] , in the combined absence of Sae2 and Sgs1. We monitored the telomere length of sae2 Δ sgs1 Δ rif2 Δ clones as described in Fig. 1 . Clones exhibited either pattern I or III ( Supplementary Fig. 4 ), but in all cases we found that telomeres were over-elongated in sae2 Δ sgs1 Δ rif2 Δ clones, similar to the rif2 Δ control cells. We concluded that not only telomerase is active in sae2 Δ sgs1 Δ but also it is sensitive to negative regulation by Rif2. Short telomeres improve the growth of the sae2 Δ sgs1 Δ cells The yKu complex controls telomere length and DNA end resection [45] . To separate the contribution of these functions in the rescue of sae2 Δ sgs1 Δ cells, we analysed the effect of the yku80-135i mutation that is defective in TLC1 binding and has short telomeres but retains telomere end protection and NHEJ function [46] . We found that the yku80–135i allele partially suppressed the slow growth phenotype of the sae2 Δ sgs1 Δ double mutant ( Fig. 5a ). Similarly, deletion of TEL1 , one key actor of telomere length maintenance, also improved growth of sae2 Δ sgs1 Δ cells ( Fig. 5b ). This effect was further enhanced when sae2 Δ sgs1 Δ tel1 Δ cells were isolated from diploid cells with very short telomeres because of deletion of both copies of TEL1 ( Fig. 5c ). A similar result was observed upon deletion of MRE11 ( Fig. 5b ).Thus, reduced telomere length appears to promote the growth of the sae2 Δ sgs1 Δ mutant. 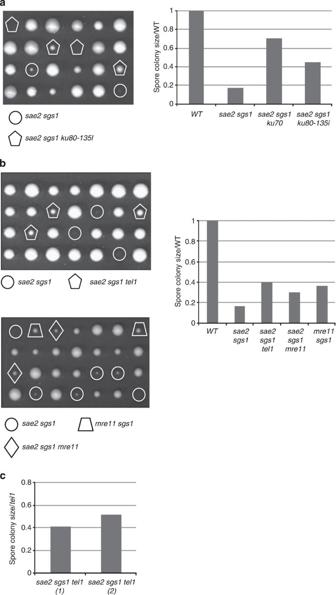Figure 5: Improved growth of thesae2Δsgs1Δ double mutant. (a) Meiotic products from asae2Δsgs1Δyku80-i135heterozygous diploid were analysed by tetrad analysis. Six representative tetrads are shown after 4 days at 30 °C. The sizes of the viable spore colonies were measured relative to WT from the same dissection plate and are plotted as mean values from two independent dissection plates. The value for thesae2 sgs1 ku70mutant is fromsupplementary Fig. 3and is shown for comparison. (b) Spore colonies fromsae2Δsgs1Δtel1Δ andsae2Δsgs1Δmre11Δ heterozygous strains. The size of the colonies was measured and plotted as described ina. (c) Atel1Δsae2Δ strain was crossed with atel1Δsgs1Δ strain. Telomeres of the resulting diploid were equilibrated before its sporulation and tetrad dissection. The graph shows mean size of the spore colonies normalized to that intel1Δ cells (1). The size of thesae2Δsgs1Δtel1Δ spore colonies inbwas normalized in the same way and plotted on the same graph for comparison (2). Figure 5: Improved growth of the sae2 Δ sgs1 Δ double mutant. ( a ) Meiotic products from a sae2 Δ sgs1 Δ yku80-i135 heterozygous diploid were analysed by tetrad analysis. Six representative tetrads are shown after 4 days at 30 °C. The sizes of the viable spore colonies were measured relative to WT from the same dissection plate and are plotted as mean values from two independent dissection plates. The value for the sae2 sgs1 ku70 mutant is from supplementary Fig. 3 and is shown for comparison. ( b ) Spore colonies from sae2 Δ sgs1 Δ tel1 Δ and sae2 Δ sgs1 Δ mre11 Δ heterozygous strains. The size of the colonies was measured and plotted as described in a . ( c ) A tel1 Δ sae2 Δ strain was crossed with a tel1 Δ sgs1 Δ strain. Telomeres of the resulting diploid were equilibrated before its sporulation and tetrad dissection. The graph shows mean size of the spore colonies normalized to that in tel1 Δ cells (1). The size of the sae2 Δ sgs1 Δ tel1 Δ spore colonies in b was normalized in the same way and plotted on the same graph for comparison (2). Full size image To address the effect of short telomeres on growth in an unbiased genetic background, we shortened telomeres in a heterozygous sae2 Δ sgs1 Δ diploid by replacing both copies of TLC1 by the doxycycline-repressible TLC1 allele ( tetO 2 -TLC1 ) [32] . After 32 PDs in the presence of doxycycline, telomere length of the diploid was reduced by about 150 bp ( Supplementary Fig. 5a ). Diploid cells treated with doxycycline and untreated controls were sporulated and dissected on Yeast extract peptone dextrose (YPD) plates. The Supplementary Fig. 5 shows the growth and telomere pattern for treated and control sae2 Δ sgs1 Δ spore clones. As expected, the doubling time of the control clones was initially longer than 4 h but decreased to about 2.5 h after approximately 45 PDs, which correlated well with abrupt telomere shortening ( Supplementary Fig. 5b,c ). In contrast, initial doubling time of the sae2 Δ sgs1 Δ clones obtained from the doxycycline-treated diploid strain was already shorter at the first time point for clones that had reduced telomere length ( Supplementary Fig. 5b,c ). The doubling time further dropped to about 2 h as cells with the shorter telomeres became enriched in liquid culture. No abrupt telomere shortening was observed in either clone. These results indicate that experimental telomere shortening independent of mutations in yKu can partially improve growth of the sae2 Δ sgs1 Δ cells. Sae2 and Sgs1 facilitate telomere replication It has been proposed that in the absence of Sae2 and Sgs1, the Ku complex prevents the processing of replication-born DSBs and hence their repair by HR [36] . Telomeres are a challenge for the replication machinery [29] rising the possibility of an increased occurrence of fork arrest and associated damage in the absence of Sae2 and Sgs1. We used neutral/neutral two-dimensional gel electrophoresis (2DGE) followed by Southern blotting to directly observe telomere replication intermediates in sae2 Δ sgs1 Δ double mutant cells grown for about 30 PDs, before telomeres abruptly shorten. More than half of the chromosome ends in S. cerevisiae contain one or two subtelomeric Y′ elements, which come in two size classes, long and short, that differ by the presence of a 1.5-kb sequence ( Fig. 6a ). We digested DNA with Cla I and used a Y′ long-specific probe as described previously [35] . Owing to the presence of tandem Y′L elements on some telomeres, two partly overlapping Y arcs corresponding to the replication of the terminal and internal Cla I fragments were observed ( Fig. 6b ). 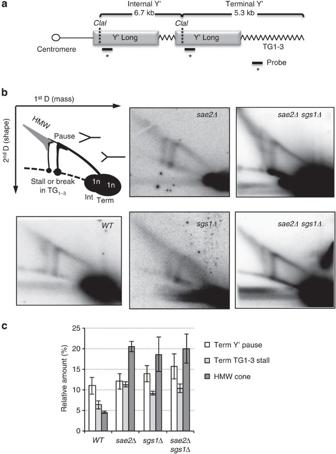Figure 6: Sae2 and Sgs1 facilitate telomere replication. (a) Schematic of a chromosome end depicting a tandem arrangement of the two long Y′ elements present at several chromosome ends, the position of theClaIsite clusters, and the Y′L-specific probe annealing site. (b) Replication intermediates at the Y′L-containing subtelomeres of the wt,sae2Δ,sgs1Δand sae2Δsgs1Δ cells visualized before abrupt telomere shortening. (c) Hybridization signals corresponding to the pause and stall of the replication fork in the terminal Y′ element, and to the HMW intermediates, as indicated in the inset tob, were normalized to the total signal from all replicating intermediates at Y′ telomeres. Mean signal values, represented as percent of total signal, for the wt (n=3),sae2Δ (n=4),sgs1Δ (n=3) andsae2Δsgs1Δ (n=7) clones are shown. Error bars represent standard error of the mean (s.e.m.).Pvalues from the paired, two-tailedt-test for the pairwise comparisons between genotypes are given in theSupplementary Fig. 6a. Figure 6: Sae2 and Sgs1 facilitate telomere replication. ( a ) Schematic of a chromosome end depicting a tandem arrangement of the two long Y′ elements present at several chromosome ends, the position of the ClaI site clusters, and the Y′L-specific probe annealing site. ( b ) Replication intermediates at the Y′L-containing subtelomeres of the wt, sae2 Δ, sgs1 Δ and sae2 Δ sgs1 Δ cells visualized before abrupt telomere shortening. ( c ) Hybridization signals corresponding to the pause and stall of the replication fork in the terminal Y′ element, and to the HMW intermediates, as indicated in the inset to b , were normalized to the total signal from all replicating intermediates at Y′ telomeres. Mean signal values, represented as percent of total signal, for the wt ( n =3), sae2 Δ ( n =4), sgs1 Δ ( n =3) and sae2 Δ sgs1 Δ ( n =7) clones are shown. Error bars represent standard error of the mean (s.e.m.). P values from the paired, two-tailed t -test for the pairwise comparisons between genotypes are given in the Supplementary Fig. 6a . Full size image We detected hybridization signal near the 2n spot (termed TG 1–3 stall; Fig. 6b ), which might reflect stalling and perhaps occasional breakage of the replication forks, which enter TG 1–3 repeats [47] . Signal intensity was stronger at this spot in either sae2 Δ and sgs1 Δ single or double mutant s compared with WT ( Fig. 6b,c and Supplementary Fig. 6a ). In addition, a blurred cone-shaped signal extending from the Y arc apex (termed high-molecular weight (HMW) cone) was visible ( Fig. 6b ). The extension of signal in the HMW range could be explained by a failure of Cla I to cut at the newly replicated arm(s) of the Y molecules because of the presence of the single-strand DNA (ssDNA) gaps [48] , [49] , [50] . The HMW cone-shaped signal was increased in the sae2 Δ and sgs1 Δ single and in the double sae2 Δ sgs1 Δ mutants as compared with WT ( Fig. 6b,c and Supplementary Fig. 6a ). The blurred appearance of the cone signal likely reflects the heterogeneity and complexity of the branched HMW structures rich in ssDNA that are possibly formed due to defects in recombination-dependent restart of the stalled replication forks near telomeres. This assumption was corroborated by the reduction of the cone signal by about 20% after pre-treatment of the DNA with Mung Bean nuclease ( Supplementary Fig. 6b ) that specifically digests ssDNA. Importantly, the cone signal in the HMW range was not detected at the rDNA locus ( Supplementary Fig. 6c ) in either WT or mutant cells. Thus, it appears to be specific for replicating telomeres. Notably, both the signal near the 2n spot and the HMW cone-shaped signal are already increased in the single mutants without being further enhanced in the double mutant. This observation suggests that Sae2 and Sgs1 likely function at different steps of the pathway that prevents and/or resolves DNA structures arising at the stalled replication forks. Sae2 and Sgs1 decrease ssDNA level upon replication defect As 2DGE suggested that both SAE2 and SGS1 deletions contribute to a replication defect at telomeres, we tested the possibility that these cells accumulate ssDNA. To this end, we analysed the number and the distribution of RPA foci in log-phase cultures. We found that sae2 Δ cells accumulate twice the number of Rfa1-CFP foci as compared with WT cells ( Fig. 7a ). To assess ssDNA at telomeres, we scored the fraction of Rfa1 foci that co-localize with Rap1 and found that deleting SAE2 increased this fraction several fold ( Fig. 7b ). As expected from its role in resolving recombination intermediates, sgs1 Δ cells accumulated an even greater level of Rfa1 foci as compared with sae2 Δ cells, although the fraction of Rfa1 foci at telomeres was similar in both strains ( Fig. 7a,b ). Both the number and telomere co-localization of the Rfa1 foci were greatly enhanced when the two mutations were combined ( Fig. 7 ). 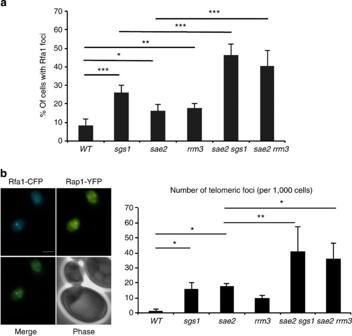Figure 7: Sae2 limits ssDNA accumulation during telomere replication. Cells of the indicated genotypes and expressingRFA1-CFPwere analysed by fluorescence microscopy. (a) The number of cells containing one or more Rfa1 foci was scored for at least three independent clones of each strain (n>300 cells for each clone). (b) The number of Rfa1 foci co-localizing with the telomeric Rap1 protein was monitored in cells expressing bothRFA1-CFPandRAP1-YFP. Errors bars indicate s.d.P-values are from the Fisher’s LSD test. *P<0,05, **P<0,01, ***P<0,0001. Scale bar=2 μm. Figure 7: Sae2 limits ssDNA accumulation during telomere replication. Cells of the indicated genotypes and expressing RFA1-CFP were analysed by fluorescence microscopy. ( a ) The number of cells containing one or more Rfa1 foci was scored for at least three independent clones of each strain ( n >300 cells for each clone). ( b ) The number of Rfa1 foci co-localizing with the telomeric Rap1 protein was monitored in cells expressing both RFA1-CFP and RAP1-YFP . Errors bars indicate s.d. P -values are from the Fisher’s LSD test. * P <0,05, ** P <0,01, *** P <0,0001. Scale bar=2 μm. Full size image A well-established function of Sae2 is associated with MRX-dependent DNA end resection at DSBs [51] . To examine whether Sae2 may also function during replication stress, the effect of SAE2 deletion was analysed in the cells lacking Rrm3, an helicase promoting replication through protein barriers [52] including telomeric and subtelomeric DNA [53] . The number of Rfa1 foci in sae2 Δ cells was strongly increased in the absence of Rrm3 ( Fig. 7a ). A fraction of these foci co-localized with RAP1 foci ( Fig. 7b ) in line with the role of Rrm3 in facilitating telomere replication. Notably, SAE2 deletion had a synthetic growth defect with Rrm3 inactivation ( Supplementary Fig. 7 ). These results suggest that Sae2 prevents ssDNA accumulation during DNA replication, and this function becomes particularly important in the absence of either Sgs1 or Rrm3. Sae2 and Sgs1 accelerates replicative senescence As we found that Sae2- and Sgs1-dependent telomere resection is dispensable for telomerase action, we sought to reveal its role in telomerase-negative cells. est2 Δ and est2 Δ sae2 Δ mutants were isolated from a heterozygous diploid strain. Cells were transferred from the dissection plate to liquid medium after about 30 PDs and serially diluted to 10 5 cells per ml every 24 h after measuring cell density. In this assay, est2 Δ cells progressively lose their growth capacity and reach crisis after 70 PDs before the appearance of survivors. The deletion of SAE2 delays the peak of senescence for about ten PDs ( Fig. 8a ), even though the starting telomere length is similar in sae2 Δ and WT cells and the rate of telomere shortening is comparable in both strains (refer to Fig. 8d ). SAE2 deletion caused even stronger delay when telomerase was turned off by adding doxycycline in the tetO 2 -TLC1 strain ( Supplementary Fig. 8 ). Therefore, Sae2 promotes generation of the signal that leads to CP activation and cell cycle arrest in the absence of telomerase. 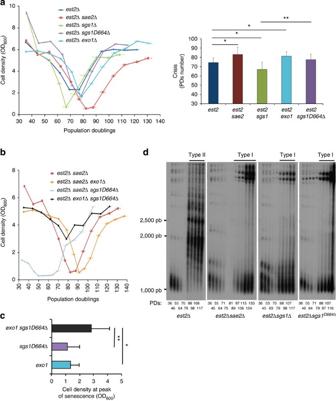Figure 8: Sae2, Sgs1 and Exo1 act in parallel to promote senescence. (a) Senescence was monitored in liquid cultures for spore colonies with the indicated genotypes. Each point represents the mean OD600value for at least four independent spores of the indicated genotypes. The mean PDs number at the peak of senescence for each strain is represented (right graph). (b) Senescence of each triple mutant was monitored in liquid cultures as ina. The data of theest2Δsae2Δ double mutant from (a) were added to facilitate comparisons. (c) Comparison of mean cell densities at the peak of senescence ofest2Δexo1Δsgs1D664Δ mutant cells withest2Δexo1Δ andest2Δsgs1D664Δ cells. (d) TG1–3probed Southern blots ofXho1-digested genomic DNA from representative clones shown ina.P-values were obtained by Fisher’s LSD test. *P<0,05, **P<0,01. Error bars indicate s.d. (est2Δ, n=8;est2Δsae2Δ,n=5,est2Δexo1Δ, n=5;est2Δsgs1Δ,n=4;est2Δsgs1D664Δ,n=10;est2Δsae2Δexo1Δ, n=6,est2Δexo1Δsgs1D664Δn=4,est2Δsae2Δsgs1D664Δ,n=8). Figure 8: Sae2, Sgs1 and Exo1 act in parallel to promote senescence. ( a ) Senescence was monitored in liquid cultures for spore colonies with the indicated genotypes. Each point represents the mean OD 600 value for at least four independent spores of the indicated genotypes. The mean PDs number at the peak of senescence for each strain is represented (right graph). ( b ) Senescence of each triple mutant was monitored in liquid cultures as in a . The data of the est2 Δ sae2 Δ double mutant from ( a ) were added to facilitate comparisons. ( c ) Comparison of mean cell densities at the peak of senescence of est2 Δ exo1 Δ sgs1 D664 Δ mutant cells with est2 Δ exo1 Δ and est2 Δ sgs1 D664 Δ cells. ( d ) TG 1–3 probed Southern blots of Xho1 -digested genomic DNA from representative clones shown in a . P -values were obtained by Fisher’s LSD test. * P <0,05, ** P <0,01. Error bars indicate s.d. ( est2 Δ , n =8; est2 Δ sae2 Δ, n =5, est2 Δ exo1 Δ , n =5; est2 Δ sgs1 Δ, n =4; est2 Δ sgs1 D664 Δ, n =10; est2 Δ sae2 Δ exo1 Δ , n =6, est2 Δ exo1 Δ sgs1 D664 Δ n =4, est2 Δ sae2 Δ sgs1 D664 Δ, n =8). Full size image The SAE2 deletion also impacts on the type of telomerase-independent survivors produced by HR. Type I survivors are generated at higher frequency compared with type II survivors, but the latter take over the culture because of their faster growth [54] . sae2 Δ est2 Δ clones were found to produce type I survivors, characterized by the amplification of both long and short Y′ subtelomeric sequences ( Fig. 8d ). Thus, Sae2 participates in the Rad59- and MRX-dependent recombination pathway that leads to the generation of type II survivors. SGS1 deletion is known to accelerate the onset of senescence in est2 Δ cells [33] . We asked whether the function of Sgs1 in the resolution of telomere recombination intermediates in presenescent cells [35] could mask its role in the resection of eroded telomeres. To address this possibility, we used the sgs1 D664 Δ separation of functions allele [55] . This allele has a defect in the processivity of resection at DSBs [56] , [57] . In agreement with previous report [33] , we found that full deletion of SGS1 accelerated the loss of viability of est2 Δ cells, although the defect was less pronounced in our strain background ( Fig. 8a ). In contrast, the sgs1 D664 Δ allele had an opposite effect, delaying the peak of senescence ( Fig. 8a and Supplementary Fig. 8 ). Assuming that sgs1 D664 Δ allele is proficient in the resolution of telomere recombination intermediates but defective in resection [57] , these results indicate that Sgs1 also contributes to resection of eroded telomeres. Noteworthy, although it has an opposite effect on the kinetics of senescence, the sgs1 D664 Δ allele impaired the formation of type II survivors as did the full deletion of the gene [33] ( Fig. 8d ), highlighting the role of the Sgs1 resection function for survivors’ formation. Introduction of the sgs1 D664 Δ mutation in exo1 Δ est2 Δ cells did not further delay senescence but dramatically attenuated the peak of senescence ( Fig. 8b,c ). In contrast, EXO1 and SAE2 deletions had additive effect on the kinetics of senescence. Surprisingly, the sae2 Δ sgs1 D664 Δ cells started to senesce in less than 40 PDs without telomerase activity. However, this phenotype most probably is related to non-telomeric defects as this strain grows very poorly even in the presence of telomerase. In agreement with data obtained in a telomere healing assay [17] , our results suggest that Exo1 and Sgs1 act through redundant pathways to generate long ssDNA at eroded telomeres but neither one can compensate for Sae2. To further evaluate the role of Sae2 in processing telomeric ends before extensive resection, we investigated its genetic interaction with capping proteins. The SAE2 deletion was introduced in rif2 Δ est2 Δ and ku80 Δ est2 Δ cells. RIF2 deletion dramatically accelerates replicative senescence because of precocious accumulation of telomeric ssDNA [58] , [59] . The deletion of SAE2 partially rescued the growth defect of rif2 Δ cells in the absence of telomerase ( Fig. 9a ). Although we cannot rule out that SAE2 and RIF2 deletions have additive independent effects, this result is in line with the role of Rif2 in regulating the function of MRX/Sae2 in resection [60] . In this case, premature senescence of the rif2 Δ sae2 Δ est2 Δ triple mutant as compared with the sae2 Δ est2 Δ double mutant would suggest that Sae2 is not the only activity inhibited by Rif2. As expected [20] , inactivation of yKu80 dramatically accelerated senescence ( Fig. 9b ) with most of the clones already senescing on the dissection plate. Remarkably, premature senescence of ku80 Δ est2 Δ cells, in contrast to that of rif2 Δ est2 Δ, was not reversed by the additional deletion of SAE2 . The latter observation supports the idea that Sae2 becomes dispensable for resecting telomeres when they are not bound by yKu. 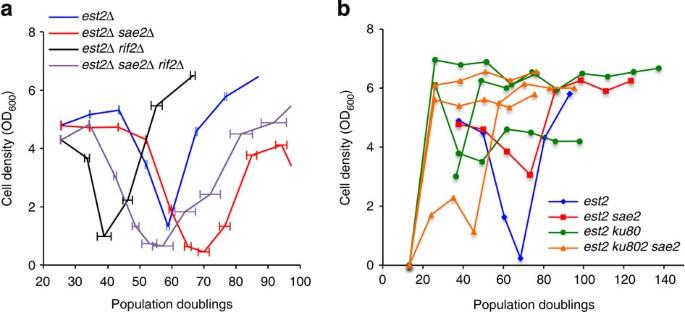Figure 9: Distinct effects ofsae2Δ inrif2Δest2Δ andku80Δest2Δ. (a) Senescence of spore colonies was monitored as described inFig. 8. Error bars indicate s.d. (est2Δ, n=5;est2Δsae2Δ,n=6;est2Δrif2Δ,n=3;est2Δsae2Δrif2Δ, n=5). (b) The senescence profile of eachest2 ku80Δ andest2 ku80Δsae2Δ spore clone is shown individually. The curves are colour-coded according to genotype.est2Δ andest2Δsae2Δ clones were isolated from the same diploid and are shown for comparison. Figure 9: Distinct effects of sae2 Δ in rif2 Δ est2 Δ and ku80 Δ est2 Δ. ( a ) Senescence of spore colonies was monitored as described in Fig. 8 . Error bars indicate s.d. ( est2 Δ , n =5; est2 Δ sae2 Δ, n =6; est2 Δ rif2 Δ, n =3; est2 Δ sae2 Δ rif2 Δ , n =5). ( b ) The senescence profile of each est2 ku80 Δ and est2 ku80 Δ sae2 Δ spore clone is shown individually. The curves are colour-coded according to genotype. est2 Δ and est2 Δ sae2 Δ clones were isolated from the same diploid and are shown for comparison. Full size image It has been proposed that Sae2 and Sgs1/Dna2 are required for the processing of native telomeres to generate the G strand overhang at each round of replication, thereby allowing telomerase recruitment [17] . A different picture emerged from our study. We demonstrated that telomeres in sae2 Δ sgs1 Δ cells can be maintained at WT length by telomerase. We explain that the short telomeres in sae2 Δ sgs1 Δ is caused by the acquisition of point mutations, notably in yKu. The fact that yKu80 mutations map to structural elements that are known to be crucial for DNA binding is consistent with the selection for yKu mutations that reduce its affinity for DNA ends. Therefore, our results are in agreement with the rescue of the sae2 Δ sgs1 Δ resection defect by allowing access of the ExoI to DNA ends [36] . Strong selection for yku mutants in the sae2 Δ sgs1 Δ background implies that yKu binding becomes the major obstacle for replication fork restart in the absence of Sae2. Intriguingly, the viability of the sae2 Δ sgs1 Δ yku Δ rad52 Δ quadruple mutant suggests that part of the rescue process is independent of recombination. Alternatively, in the absence of Rad52, forks may not end up in the same stalled configuration, precluding rescue through yKu inactivation. There is also a resection-independent component in the rescue of the sae2 Δ sgs1 Δ slow growth. Noteworthy, we found that the yku80-135i allele partially suppressed the slow growth phenotype of the sae2 Δ sgs1 Δ double mutant suggesting that short telomeres per se facilitate the phenotypic suppression of the double mutation. The absence of either Mre11 or Tel1 also improved growth of the sae2 Δ sgs1 Δ cells, but this effect could be mediated primarily by an attenuation of the CP response activated in the absence of Sae2 and Sgs1. Such Mre11/Tel1-dependent CP activated in response to unresected DSB was previously described in yeast lacking Mec1 (refs 61 , 62 ). Nevertheless, prior telomere shortening further improves the growth of the sae2 Δ sgs1 Δ tel1 Δ spore colonies highlighting the role of telomere length in sae2 Δ sgs1 Δ growth capacity. Possibly, short telomeres are weaker barriers for replication forks. Results of the 2DGE analysis of replicating telomeres are consistent with the idea that an important function of Sae2 and Sgs1 is to facilitate the completion of telomere replication. Augmentation of HMW structures in the absence of either Sae2 or Sgs1 suggests that both proteins act during the resolution of stalled forks at telomeres, likely by reducing ssDNA accumulation and avoiding engagement in inappropriate recombination events. Finally, the function of Sgs1 in yeast telomere replication is in line with the role proposed for its mammalian orthologue, the RecQ helicase Bloom, in resolving late replication intermediates at mammalian telomeres [63] . Exposure of ssDNA may be particularly undesirable at repetitive sequences, such as telomeres, which are prone to recombination. A role of Sae2 in limiting ssDNA accumulation when replication fork progression is impeded may appear contradictory with its function in association with the MRX complex in DSB resection. However, the functional relationship between MRX complex and Sae2 are not completely understood. Although the proteins act together in initiating resection [51] , Sae2 was also shown to timely remove Mre11 from DSBs [64] , [65] . Because Mre11 generates small internal gaps at stalled replication forks [66] , it is possible that Sae2 also controls the extent of Mre11-dependent degradation of nascent DNA strands at stalled forks. The ssDNA gaps created in the absence of Sae2 could be targeted by nucleases [67] . Alternatively, if not repaired, they would create single-ended DSBs at the next cycle of replication [68] . Our study therefore highlights an antagonistic relationship between the Sae2 and MRX complex responsible for ssDNA generation near collapsed replication forks. We propose that Sae2 and Sgs1 act during sequential steps of the same process that prevents aberrant transitions at the paused replication forks at telomeres and other fragile sites. In the double mutant, ssDNA would accumulate at paused forks and engages in aberrant DNA structures, which would eventually generate DSBs. At this stage, repair would be largely facilitated by inactivation of yKu that binds to DSBs and blocks ExoI access. Our data on the role of Sae2 at telomeres in the absence of telomerase showed that eroded telomeres are processed similarly to DSBs with a key role of Sae2 in initiating DNA end resection. Using the sgs1 D664 Δ allele, we clarified the impact of two separable functions of Sgs1 on replicative senescence. It is required to preserve viability of presenescent cells probably through the resolution of recombination intermediates that arise at paused replication forks in telomeric regions [35] , but once the telomeres become uncapped, Sgs1 contributes to the trimming of the 5′ ends and production of the long 3′-overhangs, which induce the DNA damage CP activation. The sgs1 D664 Δ mutation alone has a moderate impact on the kinetics of CP activation, delaying senescence to an extent similar to EXO1 deletion. This indicates that Exo1 and Sgs1 contribute equally to the generation of ssDNA at telomeres. Accordingly, CP activation is largely attenuated in the double exo1 Δ sgs1 D664 Δ mutant cells in the absence of telomerase as expected for a large defect in telomere resection. In this study, we show that deletion of SAE2 delays senescence, an effect further enhanced by the concomitant inactivation of Exo1. Contradictory conclusions have been drawn by two recent reports on the role of Sae2 during replicative senescence [69] , [70] . Ballew and Lundblad [69] did not detect any role of Sae2 until late senescence stage where SAE2 deletion would accelerate senescence, whereas Fallet et al. [70] reported a role of Sae2 in delaying senescence. The apparent contradiction between our results and those of Ballew and Lundblad [69] most probably stems from the different assays used in the two studies. Senescence assays in liquid culture used in this study allow shorter time course as compared with serial restreaking on plates and better distinguishes the time and the length of the senescence peak. In agreement with Ballew and Lundblad [69] , we found that the peak of senescence is indeed accentuated in sae2 Δ cells. We propose, however, that the defect in producing type II survivors rather than an increased senescence signal better explains this phenotype. Altogether, our data suggest that the role of Sae2/MRX in initiating resection is particularly critical at telomeres in telomerase-negative cells. Sae2 might be required to clip one of the capping proteins from eroded telomeres to allow long-range resection by Exo1 and Sgs1. The best candidate is the Ku complex whose inactivation accelerates senescence in an Exo1-dependent manner [20] . Consistent with this possibility the absence of Ku bypasses the requirement for Sae2. Yeast strains All strains were isogenic with W303-1A and are listed in the Supplementary Table 1 . Strains were constructed and analysed by standard genetic methods. Telomere Southern blot analysis Genomic DNA was prepared from about 8 × 10 7 cells and digested with Xho I. XhoI -cut DNA was resolved in 1.2% agarose gel and transferred onto a Hybond-N+ membrane. The DNA was hybridized with a radiolabelled DNA fragment composed of TG 1–3 repeats. Telomere length equilibration All strains analysed were freshly isolated from dissection of the appropriate heterozygous diploids. Dissection plates were grown for 5 days at 30 °C. After genotype analysis, the entire colonies from the dissection plates were transferred to 2 ml Yeast extract peptone dextrose (YPD) and grown for 48 h at 30 °C. Cultures were then serially diluted to 10 5 cells per ml every 2 days. To estimate the doubling time, the initial cultures were maintained in asynchronous growth conditions by diluting the cells each time the suspension reached a density of about 10 7 cells per ml. Shortening of the telomeres in the diploid cells Doxycycline (10 μg ml −1 , Sigma, cat. no. D9891) was added to a log-phase culture of tetO 2 -TLC1/ tetO 2 -TLC1 SAE2/sae2 SGS1/sgs1 diploid cells. The culture was maintained in log-phase conditions by diluting the cells each time the suspension reached a density of about 10 7 cells per ml. Aliquots were taken about every ten PDs for telomere length analysis. An aliquot of the cell culture was washed with water and immediately plated on sporulation medium at each time point. Based on telomere length analysis, dissection was performed on cells treated for 32 PDs along with the same diploid without doxycycline treatment as a control. Entire colonies of sae2 Δ sgs1 Δ cells from the dissection plates were transferred to 2 ml YPD and analysed as described above for telomere length and PD time. Senescence analysis Senescence of tetO2-TLC1 derivative strains was induced by adding 10 μg ml −1 doxycycline to exponentially growing cultures. The culture was maintained in log-phase conditions by diluting the cells each time the suspension reached a density of about 10 7 cells per ml. Using the EST2 deletion, each senescence assay started from the appropriate heterozygous diploid that was first propagated for at least 50 PDs to ensure that telomeres reached a stable equilibrium length. After 2–3 days of growth at 30 °C, the entire spore colonies were transferred to 2 ml liquid YPD to estimate the number of PDs and the suspension immediately diluted to 10 5 cells per ml. Cells were serially passaged in liquid YPD medium at 24-h intervals. For each passage, the cell density in each culture was determined and the cultures diluted back into fresh YPD medium at a cell density of 10 5 cells per ml. yKU sequencing and cloning yKU70 and yKU80 genes, including ~500 bp of 5′- and ~200 bp of 3′ UTR, were PCR amplified from the indicated strains using 5′-GATACTGGATCCGGTGCAAAACCGGATGCTC-3′ and 5′-TAGTTGGCGGCCGCAACGTTTAGCACGACAAAAGTTC-3′ as primers for yKU70 and 5′-ATAAAACTCGAGCTCAACATATAAGAATACAAGCTG-3′ and 5′-AAAGGAGCGGCCGCAACCTGCATGGCTAGTGTT-3′ for yKU80 . PCR products were sequenced by Cogenics (Beckman Coulter Genomics) and overlapping reads were assembled into contigs using SeqMan module of DNASTAR. WT and mutant genes were cloned in pRS316 as Xho I -Not I fragments. The cloned fragments were checked by sequencing for the absence of additional mutations. Telomere sequence analysis The telomere TEL01L was amplified by PCR as described [35] , [43] . PCR products treated for 5 min at 72 °C with a non-proofreading Taq polymerase were separated on 2% agarose gel and 400–500 bp fragments were purified and cloned into TA-cloning vector (InVitrogen). Because the telomere TEL01L PCR also amplified another unidentified telomere, the clones containing TEL01L were subsequently selected using a second set of specific subtelomeric primers before sequencing. Sequencing was performed by Cogenics (Beckman Coulter Genomics). Telomere sequences were aligned using Geneious software (version 6.0.5) created by Biomatters, available from http://www.geneious.com/. Conserved sequences were defined when perfectly matching to the consensus and upon single point mutation or single base deletion/insertion that next realigned with the consensus according to Lee et al. [35] The point of divergence was defined when the sequence could not be aligned anymore with the consensus sequence. Two-dimensional-gel electrophoresis DNA was purified from 10 9 log-phase cells. Briefly, after treatment with 0.1% sodium azide to preserve the replication intermediates, cells were resuspended in spheroplasting buffer (1 M Sorbitol, 100 mM EDTA, 100 U ml −1 Zymolyase T100, β-MercaptoEthanol). Pellets were washed and treated with RNase and proteinase K in buffer containing 2% CTAB (hexadecyltrimethylammonium bromide) and 1.4 M NaCl. DNA was gently extracted with chloroform/isoamyl alcohol (24:1) and precipitated via dilution to decrease salt concentration below 0.5 M. At room temperature, DNA precipitates in the presence of CTAB when NaCl concentration is below 0.5–0.7 M. DNA-CTAB precipitate was then recovered by centrifugation (10 min at 9,000 g), and dissolved in the high-salt buffer to release DNA from CTAB, precipitated with two volumes of ethanol and washed with 70% ethanol to remove residual CTAB and salt. Ten micrograms of purified DNA were digested with Cla I and subjected to neutral/neutral 2DGE to resolve replication intermediates as described [35] . DNA was then transferred on Hybond N+ membrane using standard Southern blot procedure, and hybridized with radioactively labelled Y′L-specific probe. The signal was acquired using phosphorimager, and unadjusted images were quantified in ImageQuant v5.2. To analyse the presence of ssDNA in replication intermediates, DNA was treated with Mung bean nuclease at 0.5 U μg −1 DNA for 20 min at 30 °C. A control sample was incubated in the Mung bean nuclease digestion buffer under the same condition but without the enzyme. Microscopy For fluorescent microscopy, cells from freshly dissected spore colonies were grown at low density overnight at 30 °C on YPD plates supplemented with adenine (6 mg ml −1 ). Observations were performed using a Nikon Eclipse Ti microscope with a × 100 objective. Cell images were captured with a Neo sCMOS Camera (Andor). For each field of cells, 15 images were obtained at 0.250 μm intervals along the Z -axis to allow analysis of all focal planes of each cell. Rfa1-CFP/Rap1-YFP co-localization experiments were performed on at least three independent clones of each genotype. 50–100 Rfa1 foci were analysed for each clone. Images were analysed with the NIS-AR software and subsequently exported into Adobe PhotoShop CS2 for figures preparation. Statistics Statistical analyses were performed using Fisher’s least significant difference (LSD) tests after the null hypothesis of equal means has been rejected using the analysis of variance test. Otherwise, paired Student’s t -tests were used. Sample sizes were chosen to minimize the margin of error of the mean to 10% for the significance level 0.05. How to cite this article: Hardy, J. et al. Sgs1 and Sae2 promote telomere replication by limiting accumulation of ssDNA. Nat. Commun. 5:5004 doi: 10.1038/ncomms6004 (2014).